Maternal control of suspensor programmed cell death via gibberellin signaling 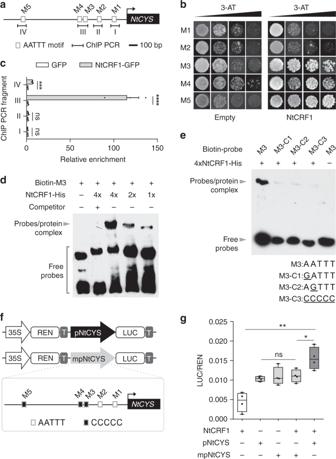Fig. 1 NtCRF1 binds to theNtCYSpromoter.aDistribution of AATTT motifs (M) in the promoter region (−1.4 kb) ofNtCYS. Fragments I (−189 to −83 bp), II (−396 to −296 bp), III (−609 to −476 bp), and IV (−1300 to −1211 bp) were subjected to ChIP-qPCR.bYeast one-hybrid assay of the interaction of NtCRF1 with M3-M5. Empty pGAD424: control.cChIP-qPCR analysis of the enrichment of NtCRF1 with the four promoter regions.pNtCRF1::GFP, control. Error bars represent the standard error (SE) of three biological replicates.dBinding of recombinant NtCRF1 to M3 was outcompeted by purified NtCRF1 (2 and 4×) and biotin-labeled DNA fragments.eTop: Binding of NtCRF1 to M3 mutants was reduced; Bottom: The sequences of M3 and the three mutant motifs.fStructure of thepNtCYS-driven andmpNtCYS(mutant promoter)-driven Dual-Luc reporter gene. 35S promoter (white arrow),pNtCYS(black arrow),mpNtCYS(gray arrow),Renillaluciferase (REN), firefly luciferase (LUC) and terminator (T) are indicated. Box: The mutant motifs ofmpNtCYS.gRelative reporter activity (LUC/REN) in tobacco protoplasts. The relative LUC activity was normalized to the REN activity (LUC/REN,n= 4). (Student’st-test; ns,P>0.05; *P<0.05; **P<0.01; ***P<0.001; ****P< 0.0001). The source data of the uncropped immunoblots are provided in the Source Data file Plant embryos are generated and develop in a stable and well-protected microenvironment surrounded by maternal tissue, which is vital for embryogenesis. However, the signaling mechanisms responsible for maternal tissue-to-proembryo communication are not well understood. Here, we report a pathway for maternal tissue-to-proembryo communication. We identify a DELLA protein, NtCRF1 ( NtCYS regulative factor 1), which regulates suspensor programmed cell death (PCD). NtCRF1 can bind to the promoter of NtCYS and regulate the suspensor PCD-switch module NtCYS-NtCP14 in response to gibberellin (GA). We confirm that GA 4 , as a primary signal triggering suspensor PCD, is generated in the micropylar endothelium by the transient activation of NtGA3oxs in the maternal tissue. Thus, we propose that GA is a maternal-to-proembryo communication signal that is decoded in the proembryo by a GID1-CRF1-CYS-CP14 signaling cascade. Using this mode of communication, maternal tissue precisely controls the embryonic suspensor PCD and is able to nurse the proembryo in a stage-dependent manner. Both animal and plant embryos are generated and developed in a stable and well-protected microenvironment, surrounded by maternal tissue. In animals, the maternal tissue impacts the embryonic development through various signals [1] , [2] , [3] . Recent work on the transcriptome of cells at the maternal-fetal interface in humans has shed new light on the mechanisms underlying maternal-fetal communication [4] . In plants, it is also reported that the maternal tissue, and in particular the seed coat, plays a critical role in embryonic development [5] , [6] , [7] , indicating interaction between maternal tissue and the proembryo is conserved. However, we know few details of the signaling pathways for maternal tissue-to-proembryo communication. The plant proembryo consists of an embryo-proper domain and a suspensor domain. The suspensor is necessary for embryonic development and plant fertility [8] , [9] and is functionally similar to the umbilical cord of the mammalian embryo, which transports nutrients and hormones from the mother to the embryo. Thus, the suspensor is the major channel for maternal-to-proembryo communication. However, unlike the umbilical cord, which is maintained until birth and provides support throughout embryonic morphogenesis and organ differentiation, the plant suspensor degenerates at a very early stage of embryonic development. This was first discovered over a century ago; however, why and how the suspensor structure degenerates at such an early proembryonic stage is unknown. We previously confirmed that NtCYS-NtCP14 functions as a switch to control the initiation of suspensor PCD [10] , and this provides a unique opportunity and practical research model for analysis of the maternal-to-proembryo communication via the suspensor. Here, we identify a tobacco DELLA protein, NtCRF1, and confirm that it is a direct regulator of the suspensor specific PCD-switch NtCYS . We show that transiently increased GA 4 in specific maternal tissue functions as a primary signal to trigger GA downstream signaling. NtCRF1 in the suspensor responds to the maternal GA signal to promote timely suspensor PCD. Thus, we reveal a complete GA signaling cascade that mediates the cell–cell communication between maternal tissues and the proembryo, which functions as the key molecular mechanism regulating suspensor PCD. NtCRF1 binds to the NtCYS promoter Based on previous work [10] , we sought to find upstream regulators of NtCYS . We first analyzed the promoter of NtCYS using PlantPan [11] and used the transcriptome data of two-celled proembryos to select candidate transcription factor (TF)-encoding genes. We screened for candidate TFs that may interact with the NtCYS promoter and selected two homologs NtCRF1 (XP_009779842.1) and NtCRF2 (XP_009789076.1). These both contain GRAS domains that have been reported to bind AATTT motifs [12] . Five AATTT motifs were found in the region −1.4 kb upstream of ATG and were named M1–M5 (Fig. 1a ), respectively. Using yeast one-hybrid (Y1H) assays, we confirmed that the two TFs stably interacted with the AATTT motifs in the NtCYS promoter (Fig. 1b and Supplementary Fig. 1a ). By chromatin immunoprecipitation (ChIP)-qPCR we assayed the five AATTT motifs to verify that NtCRF1 binds to the NtCYS promoter, and identified the motifs that preferentially interact with NtCRF1. In the immature ovaries of a pNtCRF1::NtCRF1-GFP line, NtCRF1 bound to M3, M4 ( P < 10 −4 , Student’s t -test), or M5 ( P < 0.001, Student’s t -test), but not to M1 or M2 ( P > 0.05, Student’s t -test) in comparison with the control line ( pNtCRF1::GFP ) (Fig. 1c ). We also performed an electrophoretic mobility shift assay (EMSA) to test whether NtCRF1 directly binds to NtCYS promoter in vitro using the potential DNA-binding domain LHRI-VHIID-LHRII, according to a previous report [12] (Supplementary Fig. 1b ). Incubation of the NtCYS promoter probes, including M3–M5, with NtCRF1 LHRI-VHIID-LHRII resulted in a clear band shift (Fig. 1d and Supplementary Fig. 1c, d ). Fig. 1 NtCRF1 binds to the NtCYS promoter. a Distribution of AATTT motifs (M) in the promoter region (−1.4 kb) of NtCYS . Fragments I (−189 to −83 bp), II (−396 to −296 bp), III (−609 to −476 bp), and IV (−1300 to −1211 bp) were subjected to ChIP-qPCR. b Yeast one-hybrid assay of the interaction of NtCRF1 with M3-M5. Empty pGAD424: control. c ChIP-qPCR analysis of the enrichment of NtCRF1 with the four promoter regions. pNtCRF1::GFP , control. Error bars represent the standard error (SE) of three biological replicates. d Binding of recombinant NtCRF1 to M3 was outcompeted by purified NtCRF1 (2 and 4×) and biotin-labeled DNA fragments. e Top: Binding of NtCRF1 to M3 mutants was reduced; Bottom: The sequences of M3 and the three mutant motifs. f Structure of the pNtCYS -driven and mpNtCYS (mutant promoter)-driven Dual-Luc reporter gene. 35S promoter (white arrow), pNtCYS (black arrow), mpNtCYS (gray arrow), Renilla luciferase (REN), firefly luciferase (LUC) and terminator (T) are indicated. Box: The mutant motifs of mpNtCYS . g Relative reporter activity (LUC/REN) in tobacco protoplasts. The relative LUC activity was normalized to the REN activity (LUC/REN, n = 4). (Student’s t -test; ns, P > 0.05; * P < 0.05; ** P < 0.01; *** P < 0.001; **** P < 0.0001). The source data of the uncropped immunoblots are provided in the Source Data file Full size image As M3 was the major binding site, we performed a competition assay using unlabeled M3 probe. The binding of NtCRF1 LHRI-VHIID-LHRII to M3 was obviously reduced by the unlabeled M3 probe, further confirming the binding between NtCRF1 LHRI-VHIID-LHRII and M3. We also mutated the AATTT motif in M3 to GATTT, AGTTT, or CCCCC (Fig. 1e ); this greatly reduced the binding of NtCRF1 LHRI-VHIID-LHRII to the promoter fragments (Fig. 1e ). A deletion derivative of NtCRF1 (LHRI-VHIID-LHRII) bound to M3, but not to the mutants, indicating that the LHRI-VHIID-LHRII domain is responsible for recognition of the AATTT motif (Fig. 1e ). NtCRF2 yielded similar results (Supplementary Fig. 1e, f ). To test whether NtCRF1 can activate expression of NtCYS , we utilized a dual luciferase assay based on transient transcription in protoplasts of Nicotiana benthamiana (Fig. 1f ) and examined the effect of NtCRF1 expression on NtCYS promoter activity. As shown in Fig. 1g , transiently expressed NtCRF1 obviously promoted NtCYS expression in the protoplasts. In addition, we created a mutant pNtCYS , in which the AATTT motif in M3–M5 was replaced by CCCCC. The result confirmed that induction of NtCYS by NtCRF1 depended on the AATTT motif in M3–M5 (Fig. 1f, g ). To gain insight into the spatiotemporal expression pattern of NtCRF , we generated transgenic plants carrying the pNtCRF1::NtCRF1-GFP or pNtCRF2::NtCRF2-GFP constructs. We observed that NtCRF1 was widely expressed in various tissues (Supplementary Fig. 2 ). In proembryos, NtCRF1-GFP and NtCRF2-GFP were detected in both basal and apical cell lineages, confirming expression of both NtCRF1-GFP, NtCRF2-GFP and NtCYS-GFP [10] in the basal suspensor cell (SC) (Fig. 2a and Supplementary Fig. 3a ). We also observed that NtCRF1-GFP fluorescence intensity was high in the basal cell lineage ( P > 0.05 compared to stage 1, Student’s t -test) until stage 2, sharply declined at stage 3 ( P < 10 −4 compared to stage 2, Student’s t -test), and was scarcely detectable at stage 4 ( P < 10 −4 compared to stage 3, Student’s t -test) (Fig. 2b ). These changes in expression coincided with those of NtCYS-GFP [10] . Therefore, NtCRF1 may positively regulate the expression of NtCYS in the basal SC. Fig. 2 NtCRF1 promotes NtCYS expression and suppresses PCD in basal cells. a Localization of NtCRF1-GFP during early embryogenesis in pNtCRF1::NtCRF1-GFP plants. Magnified images of corresponding basal SCs are shown below. b Relative fluorescence intensity of NtCRF1-GFP in basal SCs ( n = 16–31). c CRISPR/Cas9-mediated targeted mutagenesis of NtCRF1 . Top: Schematic of NtCRF1 showing the CRISPR/Cas9 target site (arrow). Bottom: Alignment of the sequences showing the insertion or deletion sites (red); numbers, translated amino acids (aa). d Expression of NtCYS was reduced in the crf1 mutants. e Expression of NtCYS is increased in the pNtCRF1::NtCRF1-GFP line ( OE-NtCRF1 ). (Two-way ANOVA, ** P < 0.01). f Nuclear DNA fragmentation in two-celled proembryos of WT and crf1.1 . g Frequency of two-celled proembryos with TUNEL-positive basal cells in WT and crf1 ( n = 98–109). h Frequency of aborted seeds in WT and crf1 lines ( n = 200–300 seeds per line). i Abnormal suspensors (stars indicated) in crf1 lines by modified pseudo-Schiff-propidium iodide (PI) staining. Data are the means ± SE of 3 independent experiments in e , g and 5 independent experiments in d , h (Student’s t -test, * P < 0.05, ** P < 0.01, *** P < 0.001). Scale bars: 10 μm ( a , f ), 20 μm ( i ). The source data of the graphs are provided in the Source Data file Full size image NtCRF1 regulates NtCYS expression and induces suspensor PCD To evaluate potential regulatory functions and roles in suspensor PCD, we silenced NtCRF1 using an independent RNA interference (RNAi) construct expressed under the native promoter and selected six homozygous RNAi lines for further analysis (Supplementary Fig. 4a–c ). Because NtCRF2 mutants (Supplementary Fig. 3b ) showed no seed development phenotypes (Supplementary Fig. 3c, d ) and no effects on NtCYS expression (Supplementary Fig. 3e ), we subsequently focused on NtCRF1 . We analyzed the expression level of NtCYS in 5-DAP seeds (5 days after pollination; Stage 2) to assess the influence of NtCRF1 downregulation on NtCYS expression. The expression level of NtCYS was significantly reduced in the NtCRF1-RNAi lines (Supplementary Fig. 4c ). To exclude any off-target effects of RNAi, we generated Ntcrf1 mutants using the CRISPR/Cas9 system (Fig. 2c ). As expected, the expression level of NtCYS was significantly reduced in the mutants ( P < 0.01, Student’s t -test) (Fig. 2d ). In addition, we determined the expression levels of NtCYS in NtCRF1 overexpression lines ( pNtCRF1::NtCRF1-GFP ) which had significantly greater NtCYS expression ( P < 0.01, Two-way ANOVA) (Fig. 2e ), indicating that NtCRF1 promotes the expression of NtCYS and is likely involved in regulating suspensor PCD. Next, we evaluated nuclear DNA integrity in the early proembryos of wild type (WT), NtCRF1-RNAi , and Ntcrf1 lines using the terminal deoxynucleotidyl transferase dUTP nick-end labeling (TUNEL) technique. In WT plants, the TUNEL signal first appeared in the suspensor at stage 4 (32-celled embryo) [10] . However, in the NtCRF1-RNAi and Ntcrf1 mutant lines, the TUNEL signal was detected at the two-celled proembryo stage (Fig. 2f, g and Supplementary Fig. 4d, e ). Moreover, 10–29% of embryos in NtCYS-RNAi seeds aborted (Supplementary Fig. 4f–h ), as did about 28% of those in Ntcrf1 mutant seeds (Fig. 2h ). Notably, the suspensor of the aborted embryos showed abnormal morphology (Fig. 2i and Supplementary Fig. 4f ). Due to precocious PCD, the basal cell lineage stopped dividing and degenerated. Thus, these abnormal proembryos were generally without suspensor. As an obvious phenotype, disorganized cell division was observed in all of these abnormal embryos. Pattern formation was disturbed and proembryo development was arrested at early stages. In some of the abnormal proembryos, suspensor structure could still be observed. In fact, although PCD was initiated at stage 1 in most of the proembryos, it could also occur at stage 2 or 3 in the rest of the proembryos. Thus, suspensor-like structures could be still generated in these abnormal proembryos (Supplementary Fig. 4f ). In addition, we also tested the expression of NtCYS by qRT-PCR in pNtCRF1::NtCRF1-GFP lines at stage 2 (Fig. 2e ). Although the mRNA level of NtCRF1 was increased (Supplementary Fig. 5a ), NtCRF1-GFP soon disappeared at stage 4 (Fig. 2a ). In this case, the expression of NtCYS showed no notable change at stage 4 (Supplementary Fig. 5a ) and thus, the PCD initiation occurs normally as in WT (Supplementary Fig. 5b, c ). These data suggest that NtCRF1 suppresses PCD by promoting NtCYS expression during normal suspensor development. This anti-cell-death role of NtCRF1 is indispensable for the formation of a functional suspensor and normal embryogenesis. NtCRF1 functions as a DELLA protein in early embryogenesis Sequence analysis suggests that NtCRF1 is a member of the DELLA family (Supplementary Fig. 6 ). Most DELLA proteins can bind to the GA receptor GIBBERELLIN-INSENSITIVE DWARF 1 (GID1) in the presence of bioactive GA [13] . After binding to GA-GID1, DELLA proteins are rapidly degraded [14] . To determine whether NtCRF1 responds to GA, we examined NtCRF1-GFP fluorescence in the basal cell of two-celled proembryos of the pNtCRF1::NtCRF1-GFP line. After GA 4 treatment, NtCRF1-GFP fluorescence was significantly reduced (Fig. 3a, b ), indicating the degradation of NtCRF1. Furthermore, treatment of 4-DAP seeds of pNtCRF1::NtCRF1-GFP line with the GA biosynthesis inhibitor paclobutrazol (PAC) resulted in the maintenance of the NtCRF1-GFP signal until stage 5, whereas in control, the NtCRF1-GFP signal was not detected at this stage (Fig. 3c ). These data suggest that NtCRF1 responds to GA and may play a role in GA signaling during suspensor PCD. Fig. 3 GA induces suspensor PCD via the NtCRF1-NtCYS pathway in vitro. a NtCRF1-GFP fluorescence in response to GA 4 in four-celled proembryos. 0.05% ethyl alcohol as control. b NtCRF1-GFP fluorescence in the basal cells of two-celled proembryos during treatment with GA 4 (or ABA) ( n = 9). c NtCRF1-GFP in embryos derived from two-celled proembryo in cultured seeds after 72-h treatment with PAC. d Quantification of GA 15 , GA 9 , GA 4 , and GA 51 in WT seeds at stages 1, 3, and 5 (pg per 1000 seeds, ± SE). e Cultured embryos stained with fluorescein diacetate (FDA), PI, and TUNEL. f Frequency of cultured embryos with PI-positive basal cells ( n = 128–152). g Frequency of treated cultured embryos with TUNEL-positive basal cells ( n = 106–126). h qRT-PCR analysis of NtCYS expression in 4-DAP seeds after treatment for 12-h with 100 μM ABA, PAC, or GA 4 . Data are the means ± SE of three independent experiments (Student’s t -test; ns, P > 0.05; ** P < 0.01; **** P < 0.0001). Scale bars: 10 μm. The source data of the graphs are provided in the Source Data file Full size image To confirm the role of NtCRF1 in GA signaling, we found all seven NtGID1 genes in tobacco genome [15] (Supplementary Fig. 7a ). We found evidence that four were expressed in two-celled proembryos (Supplementary Fig. 7b ). NtGID1B and NtGID1B2 were not found in the two-celled promembryo RNA-seq dataset. Next, by yeast two-hybrid (Y2H) assay we confirmed that, in the presence of bioactive GA, NtCRF1 interacts with NtGID1B3 (XP_016477564.1), NtGID1B5 (XP_016489970.1), and NtGID1C2 (XP_016494194.1) GA receptors, respectively (Supplementary Fig. 7c). Furthermore, these three NtGID1 s were expressed in the suspensor of a 32-celled embryo, the stage at which suspensor PCD is triggered (Supplementary Fig. 7d ). To further confirm that NtCRF1 functions as a DELLA protein, we observed seedling development in both the NtCRF1 overexpression line L8 ( p35S::NtCRF1-GFP ) (Supplementary Fig. 8a ) and Ntcrf1.1 mutant. We found that L8 showed shorter hypocotyls (Supplementary Fig. 8b, c ), whereas Ntcrf1.1 showed longer hypocotyls. The phenotype of hypocotyl was attributed to a change in cell length, rather than cell number (Supplementary Fig. 8d-f ). Furthermore, we demonstrated that these plants have altered responses to GA and PAC treatment, indicating a role of NtCRF1 in GA-induced hypocotyl growth, similar to that of known DELLAs (Supplementary Fig. 8g-j ). In addition, we expressed NtCRF1-GFP and ( crf1 -Δ17)-GFP, without the DELLA domain, in tobacco BY-2 cells. We found that the GFP fluorescence in the nuclei of the BY-2 cells expressing ( crf1 -Δ17)-GFP was not affected by GA treatment, whereas nuclear fluorescence was not detectable in the BY-2 cells expressing NtCRF1-GFP after the same GA treatment (Supplementary Fig. 8k ). Therefore, these data confirm that NtCRF1 functions as a DELLA protein and participates in the GA signaling pathway during early embryogenesis. GA as a primary signal induces suspensor PCD Based on above results we hypothesized that GA is a primary signal that triggers suspensor PCD via NtCRF1. Therefore, we first investigated whether endogenous bioactive GA 1 or GA 4 are present in WT seeds at stage 1, 3 (prior to suspensor PCD), and 5 by ultra-performance liquid chromatography tandem mass spectrometry (UPLC-MS/MS). We detected GA 4 , but not GA 1 , before suspensor PCD (Fig. 3d and Supplementary Fig. 9a ), suggesting that GA 4 triggers suspensor PCD. Then, using our embryo culture system [16] , we tested whether GA 4 is capable of inducing suspensor PCD. We cultured two-celled proembryo cells with exogenous GA 4 or abscisic acid (ABA; control). Approximately 36% of the cultured proembryos had propidium iodide (PI)-positive and fluorescein diacetate (FDA)-negative SCs after 72-h (stage 3) ( P < 0.01 compared to ABA or 0.05% ethyl alcohol, Student’s t -test), indicating that GA 4 induces SC death (Fig. 3e, f ). To confirm this finding, we evaluated nuclear DNA integrity in GA 4 -treated proembryos by TUNEL within 48-h (stage 2). In addition, the NtCYS expression was also decreased within 12-h (Fig. 3h ) ( P < 0.01 compared to 0.05% ethyl alcohol, Student’s t -test). The suspensors of 25% of proembryos were TUNEL-positive (Fig. 3e, g ). We further tested the suspensor PCD when GA biosynthesis was inhibited by PAC treatment at stage 4. We found that the PCD delayed and the suspensor cells could continue dividing at the stage (Supplementary Fig. 10 ). Therefore, it is clear that GA 4 as a signal induces suspensor PCD via the NtCRF1-NtCYS pathway. To examine how the timing of bioactive GA accumulation may be controlled, we investigated the dynamic distribution of bioactive GA. GA3ox, a GA oxidase, catalyzes the final step of the pathway to produce GA 1 and GA 4 . Its activity is therefore indicative of GA synthesis and distribution [17] . Thus, we cloned all homologous GA3ox genes expressed in seeds before suspensor PCD, including the known NtGA3ox1 (AB032198) and NtGA3ox2 (EF471116) genes, and a homologous GA3ox gene, named NtGA3ox3 (XP_016453191.1) (Supplementary Fig. 11 ). We examined the expression of these NtGA3oxs in seeds. Interestingly, expression of the three NtGA3ox genes peaked prior to initiation of suspensor PCD (stage 4) (Fig. 4a ) and remained at a low level thereafter. This expression pattern of key bioactive GA synthesis genes suggests a transient increase in the level of bioactive GA in seeds immediately before stage 4, which may trigger PCD of SCs. To confirm the above, we used nlsGPS1 [a nucleus-targeted variant of gibberellin perception sensor 1 (GPS1)] as a bioactive GA sensor in vivo [18] . We generated stable transgenic lines expressing pL25::nlsGPS1. L25 was demonstrated as a reference gene with high expression stability [19] and wide expression in vegetative tissues and seed including seed coat, endosperm, and embryo. We assessed the relative bioactive GA content by calculating the nlsGPS1 emission ratios. The results showed that the level of bioactive GA was significantly increased ( P < 10 −4 , Student’s t -test) at stage 3 compared to that at stage 1 (Fig. 5a, b ), in agreement with the NtGA3oxs expression (Fig. 4a ) and GA 4 content data (Fig. 3d ). Thus, immediately before suspensor PCD, NtGA3oxs expression is upregulated, and GA 4 is therefore transiently increased, which degrades NtCRF1 and triggers suspensor PCD. Fig. 4 Bioactive GA biosynthesis during early embryogenesis. a qRT-PCR analysis of NtGA3ox1 , NtGA3ox2 and NtGA3ox3 expression; GAPDH was used as the internal control. b Expression of genes related to GA biosynthesis [ NtGA20ox1 ( Ntc12 , AB012856.1) and NtGA20ox2 ( Ntc16 , AB016084.1)], deactivation [ NtGA2ox1 (AB125232.1), NtGA2ox1-like (XM_016586923.1), NtGA2ox3 (EF471117), and NtGA2ox5 (EF471118)], and signaling in WT two-celled proembryos (stage 1) via transcriptome analysis, and via qRT-PCR analysis in WT four-celled proembryos (stage 2). GAPDH was used as the internal control. Values are means ± SE of three biological replicates. nd, not detected. c Expression of NtGA3ox1 and NtGA3ox3 during embryogenesis. d Expression of NtGA3ox2 and NtGA3ox3 in the developing seed coat. Asterisks, micropylar ends; Scale bars: 10 μm ( c ), 100 μm ( d ). The source data of the graphs are provided in the Source Data file Full size image Fig. 5 Transient increase in, and polar distribution of, bioactive GA in seeds. a Left: Images of the nlsGPS1 emission ratios of unfertilized (UF), 4-DAP and 6-DAP seeds. Right: Images of the nlsGPS1 emission ratios of an optical section of a 4-DAP or 6-DAP seed. Boxes: micropylar endothecium. b Box plot of the nlsGPS1 emission ratios of the whole seed coat ( n > 46 nuclei). c nlsGPS1 emission ratios of the micropylar and chalaza ends [dashed lines in a ; n > 20 nuclei]. d Box plot of the nlsGPS1 emission ratios of stage 1 or 3 seeds [boxed region in a ; n > 10 nuclei]. e NtCRF1-GFP was absent from the basal SC at stage 3. Fluorescence signal intensities along a line across all SCs (red arrows). X -axis, relative GFP signal intensity (green); y -axis, relative distances along the line. Gray shading, positions of nuclei. f and g Images of the nlsGPS1 emission ratios of 4-celled and 12-celled proembryos in WT background. Data are the means ± SD (standard deviations) (Student’s t -test; ns, P > 0.05; *** P < 0.001; **** P < 0.0001). ME micropylar end, CE chalaza end. Scale bars: 100 μm ( a ), 10 μm ( e – g ). The source data of the graphs are provided in the Source Data file Full size image Maternal GA triggers suspensor PCD We next sought to investigate the specific tissue that is the source of GA 4 that triggers suspensor PCD. Because PCD occurs in basal SCs, we inferred that GA may be produced in the embryo, the surrounding endosperm cells, or the maternal tissue (i.e., the seed coat) and move to the basal SC. In two-celled and four-celled proembryos,  genes related to GA signaling were expressed, but those associated with GA biosynthesis and metabolism were not or at a quite low level (Fig. 4b ). Next, we generated three pNtGA3ox::H2B-GFP constructs to determine the location of GA synthesis. NtGA3ox1 , NtGA3ox2 , and NtGA3ox3 were not expressed in the endosperm and proembryo of the transgenic lines before stage 3 (Fig. 4c, d and Supplementary Fig. 9c, d ). Furthermore, the three NtGA3oxs were not expressed in the suspensor of a 32-celled embryo, the stage at which suspensor PCD is triggered (Supplementary Fig. 9b ). However, these genes were expressed in the seed coat and towards the micropyle region up to stage 4 (Fig. 4d and Supplementary Fig. 9d ). This suggests that the GA 4 that triggers PCD likely originates from maternal tissue, particularly the micropyle part of the seed coat. Accordingly, we found that bioactive GA exhibited a polar distribution in developing seeds: the mean nlsGPS1 emission ratio increased significantly from the chalaza to the micropylar ends ( P < 10 −4 , Student’s t -test) (Fig. 5a, c ). This is in agreement with the polar activation of NtGA3oxs at the same stage (Fig. 4d and Supplementary Fig. 9d ). Furthermore, we found that bioactive GA was localized mainly to the inner layer of the seed coat, the endothelium. The bioactive GA signal arose in the micropyle pole of the endothelial layer (Fig. 5a, d ), to which the suspensor is connected. Therefore, it is clear that the bioactive GA level is transiently increased in the micropylar endothelium cells adjacent to the basal SC due to timely activation of NtGA3oxs . Thus, maternal GA likely enters the basal SC and induces the GA response. To confirm this, we analyzed active GA signaling in the pNtCRF1::NtCRF1-GFP line. Before stage 2, we observed a strong GFP signal in the basal SC, which rapidly diminished as the GA level in the micropyle endothelium increased (Fig. 5e ), indicating activation of GA signaling in the basal SC. Interestingly, the GFP signal gradually declined from the basal SC to the vertically adjacent cell (Fig. 5e ), as did the occurrence of PCD. The nlsGPS1 emission ratio indicated that bioactive GA appeared in the basal SC at stages 2 and 3 (Fig. 5f, g ), and subsequently moved to the vertically adjacent cell along with a decrease in the NtCRF1-GFP signal. This is in consistent with sequential decline of NtCRF1-GFP and occurrence of PCD. Therefore, entry to the basal cell of maternal GA triggers suspensor PCD. To further confirm the induction of suspensor PCD by maternal GA in vivo, we ectopically expressed NtGA3ox1 in the endothelium, endosperm, proembryo, and seed coat under the control of four tissue-specific promoters, respectively (Fig. 6a and Supplementary Fig. 12a ). Ectopic expression of NtGA3ox1-GFP in the seed coat, endosperm, and proembryo did not influence NtCYS expression (Supplementary Fig. 12 b–d). However, ectopic expression of NtGA3ox1-GFP in the endothelium, to which the basal SC is connected, downregulated NtCYS expression (Fig. 6b ). We also evaluated proembryo development in the pTPE8::NtGA3ox1-GFP (TG) lines. As expected, we detected PCD at the two-celled proembryo stage, as in the NtCRF1 downregulation and NtCYS - RNAi lines. The basal cells in approximately 25% of the two-celled proembryos contained TUNEL-positive nuclei (type 1), as did both cell types of around 57% of the two-celled proembryos (type 2) (Fig. 6c, d ). This basal cell PCD prevents suspensor establishment during embryogenesis (Fig. 6f ), resulting in the abortion of about 50% of seeds (Fig. 6e ). Next, we crossed the pNtCRF1::NtCRF1-GFP line with the TG-8 line to monitor the dynamics of NtCRF1 in the presence of ectopic expression of NtGA3ox1-GFP in the endothelium. As expected, NtCRF1-GFP fluorescence was absent from the four-celled and two-celled proembryos (13/24) (Fig. 6g ). Therefore, suspensor PCD is triggered, via NtCRF1, by bioactive GA from maternal endothelial cells. Fig. 6 Ectopic expression of NtGA3ox1-GFP in the endothelium triggers PCD. a Localization of NtGA3ox1-GFP in the endothelium of pNtTPE8::NtGA3ox1-GFP plant. b Increased expression of NtGA3ox1 and decreased expression of NtCYS in the TG-8 and TG-11 lines. c TUNEL test in two-celled proembryos from WT and TG-8. d Frequency of two-celled proembryos with TUNEL-positive apical and basal cells in WT and TG-8 ( n = 105–112). e Frequency of aborted seeds in WT and TG-8. ( n = 1000–1500). f PI-staining of abnormal embryos with no suspensor in the TG-8 line. g NtCRF1-GFP signal in early proembryos after crossing WT and pNtCRF1::NtCRF1-GFP (CG) lines. Data are the means ± SE of 3 independent experiments in ( b , c ) and 5 in e (Student’s t -test, * P < 0.05, ** P < 0.01, *** P < 0.001); Scale bars: 150 μm ( a ), 10 μm ( c , g ), 20 μm ( f ). The source data of the graphs are provided in the Source Data file Full size image In addition, we also tried to look at the relevant aspects in Arabidopsis. As reported, AtGA3oxs are inactive during early embryogenesis [17] . Transcriptome analysis of GA3oxs and GA20oxs also suggests that GA biosynthesis is inactive in early proembryos [20] . GA signaling activation after fertilization specifically occurs in the seed coat of Arabidopsis [21] . These data suggest that at least the location of GA biosynthesis in maternal tissue might be conserved during early embryogenesis. Thus, we further tested the influence of loss-of- DELLA function or deficient GA on the suspensor development in Arabidopsis. Indeed, the global - della mutant caused defected seeds and reduced fertility (Supplementary Fig. 13a ), similar to that previously reported [22] . Moreover, we found that abnormal cell division was triggered in the suspensors of these abortive seeds (Supplementary Fig. 13b ), suggesting that loss-of- DELLA function promotes suspensor further development instead of PCD. For genetic evidence, we attempted to use WT pollen to fertilize the GA-deficient mutant ga1-3 in Landsberg erecta (L er ) background. Unfortunately, ga1-3 mutant showed defective pistils (Supplementary Fig. 13c ) and infertile ovules (Supplementary Fig. 13d ), similar to that observed in ga1-3 in Columbia background [23] , ga1-1 [24] , and ga20ox triple mutant [23] . As a result we were unable to conclusively analyze the maternal effects of GA on suspensor PCD in Arabidopsis. In summary, we demonstrated that NtCRF1 binds to the M3 motif of the NtCYS promoter. In general, DELLA proteins do not contain classical DNA-binding domains, and thus require another TF to bind to promoter and modulate gene expression [25] , [26] . However, we found that NtCRF1 that has characteristics typical of DELLA proteins in response to GA can bind to the NtCYS promoter. Recently, a crystal structure analysis revealed that the GRAS domain of OsSCL7 binds to DNA in a dimer form [27] . We also found that NtCRF1 possesses both DELLA and GRAS domains (Supplementary Fig. 6b ), and NtCRF1 and NtCRF2 could form a homo-dimer or hetero-dimer by Y2H and that the GRAS domain of NtCRF1 may mediate its binding to the promoter of NtCYS (Supplementary Fig. 1b, g ) as AtSHR and AtSCR interact directly with the promoters [28] . Moreover, we confirmed that NtCRF1 promotes the expression of NtCYS , and degradation of the former at stage 3 reduces NtCYS expression, resulting in the activation of NtCP14 and thence suspensor PCD. Thus, maternal GA signal and proembryo responsor NtCRF1 mediate maternal-proembryo communication via the GA-GID1-CRF1-CYS-CP14 signaling cascade to precisely control the maternal-embryo connection (Supplementary Fig. 14 ). It was reported that GA could trigger tapetum PCD in flowering plants via the GAMYB transcription factor [29] , which is involved in reproductive development during land plant evolution [30] . Interestingly, we also found seven GAMYB- like genes expressed in tobacco two-celled proembryos, and thus, it is worthy to investigate the relationship between GAMYB and suspensor PCD in the near future. In fact, during land-plant evolution, the GA-DELLA regulatory mechanism arose via independent stepwise recruitment of the GA-stimulated GID1-DELLA interaction [13] . In earlier stages [~430 million years ago (MYA)], GA was not involved in the GID1-DELLA interaction. Later, GID1-DELLA interactions became susceptible to potentiation by bioactive GA during the period of the bryophyte and lycophyte divergences (~430–400 MYA) [13] . Notably, an embryonic suspensor-like structure was first generated in low plants during the same period [8] , indicating that during plant evolution the establishment of the GA-dependent GID1-DELLA interaction was coupled to that of the suspensor structure. Thus, GA signaling is likely involved in maternal tissue-to-proembryo communication as it evolved in lower plants and maternal control of the connection between maternal tissue and the embryo might be an inborn character of embryogenesis for precise control of the duration of auxin and nutrient supply, which is critical for the embryos to establish full ability for independent development before their detachment from mother plant body. Materials Arabidopsis plants were grown in 16 h light/8 h dark conditions at 20–22 °C. N. tabacum L. cv. Petite Havana SR1 tobacco plants were grown under a 16/8 h light/dark cycle at 25 °C. Ntcrf mutants were generated using the clustered regularly interspaced short palindromic repeats (CRISPR)/CRISPR-associated protein 9 (Cas9) system [31] , [32] . The CRISPR target of NtCRF was selected as described [31] , [32] , and the vectors were transferred into SR1. The genomic region surrounding the CRISPR target sites of NtCRF were amplified by PCR, and the segment was subjected to Sanger sequencing to screen for mutants. T2 plants were used for phenotyping and T-DNA was already separated away, and identified using CRISPR/Cas9 vector-specific primers. Primer sequences are listed in Supplementary Data 1 . Screening for NtCYS regulative factors Based on our previous work on transcript profiling of two-celled proembryo, we first screened all the TFs expressed in the two-celled proembryos. We found 1267 candidates that belong to 35 gene families. Then, we analyzed the promoter sequence of NtCYS via PlantPan [11] . We found five AATTT motifs in NtCYS promoter according to the report that GRAS could bind to the AATTT motif [12] . Thus, we only focused on GRAS family that expressed in the two-celled proembryos. We isolated these five motifs embedded within a 25-bp region of the surrounding promoter sequence according to the required length of a bait for Y1H [12] . Yeast one-hybrid assays Yeast one-hybrid assays were conducted using the Matchmaker One-Hybrid System (Clontech). The 25-bp AATTT region surrounding the NtCYS promoter sequences was synthesized with EcoR I and Xba I flanking restriction sites, and cloned into an EcoR I- Xba I-digested pHISi-1 bait vector. For expression in yeast, NtCRF1 , NtCRF2 , and other TF cDNAs were cloned into the pGAD424 prey vector. Saccharomyces cerevisiae YM4271 (Clontech) was used as the host. Transformation was confirmed by growth on SD medium containing 0, 15, 30, or 60 mM 3-AT (a competitive inhibitor of the His3 gene product) (A8056; Sigma). The primers used are shown in Supplementary Data 1 . Yeast two-hybrid assays Yeast two-hybrid assays were performed according to the manufacturer’s protocol (Clontech). Briefly, S . cerevisiae strain AH109 was transformed with the bait construct pGBKT7-NtGID1s and subsequently with pGADT7-NtCRF1. Vectors lacking coding region insertions were used as negative controls. Protein interactions were scored based on growth on defined synthetic medium lacking Trp, Leu, His, and adenine in the presence or absence of 10 μM GA 1 (G377495; TRC) and GA 4 (G7276; Sigma). The primers used are shown in Supplementary Data 1 . ChIP-qPCR analysis Pooled unfertilized ovaries (~1 g) from pNtCRF1::NtCRF1-GFP and pNtCRF1::GFP plants were cross-linked under vacuum in 1% (w/v) formaldehyde for 30 min at room temperature. Cross-linking was quenched by the addition of 0.125 M glycine and vacuum infiltration continued for a further 15 min. The cross-linked tissues were frozen in liquid nitrogen and ground to a fine powder. ChIP assays were performed using the ChIP Kit-Plants (ab117137; Abcam). Nuclei were extracted and chromatin was disrupted using an Ultrasonic Cell Disruptor (JY92-IIN; Scientz) with 10 cycles on ice (15 s each at 30% duty cycle/1 min cooling). Chromatin (150 µl) was immunoprecipitated with 4 μl of an anti-GFP antibody (ab290; Abcam) for 90 min. The purified DNA fragments were used as the template for qPCR. qPCR was performed using the FastStart Essential DNA Green Master Mix (22682700; Roche) with three technical replicates, and threshold cycle numbers (Ct) were determined using a CFX Connect Real-Time PCR Detection System (Bio-Rad). Fold enrichment of the targeted genomic sequences over IgG was calculated as: 2 −(Ct CHIP − Ct IgG ) , where Ct ChIP and Ct IgG are the mean threshold cycles of triplicate PCRs of DNA samples immunoprecipitated using an anti-GFP antibody and the control IgG, respectively. All qPCR reactions were subjected to melt curve analyses and agarose gel electrophoresis to confirm the presence of a single specific product. The qPCR primer sequences are listed in Supplementary Data 1 . Electrophoretic mobility shift assay The DNA-interaction domain of NtCRF1 (153–396 aa) and NtCRF2 (207–417 aa) was inserted into pET32a (Novagen), respectively. The resulting plasmid was transformed into Escherichia coli BL21 (DE3). The recombinant NtCRF1-His protein was expressed and purified according to the manufacturer’s instructions. The 55-bp region of the promoter sequence surrounding AATTT was synthesized and the 5′-end was biotinylated (GenScript) and dissolved in a buffer (10 mM Tris and 1 mM EDTA). EMSAs were performed using the LightShift Chemiluminescent EMSA Kit (20148; Thermofisher). The labeled oligonucleotides were added to a 20-μl reaction mixture composed of 1–4 μg of the protein extract, 20 fmol biotin end-labeled target DNA, 4 pmol unlabeled target DNA (competitor), 1× DNA binding buffer, 1 μg poly(dI-dC), 2.5% glycerol, 0.05% NP-40, 50 mM KCl, and 5 mM MgCl 2 . After incubation for 20 min at 25 °C, the reaction products were resolved in 6% native polyacrylamide gels with 0.5× TBE buffer. The blots were developed using the Chemiluminescent Nucleic Acid Detection Module Kit (89880; Thermo Scientific). The primers used are shown in Supplementary Data 1 . Transient transcription dual-luciferase assay The reporters were constructed based on pGreenII 0800-LUC vector [33] and the effectors were constructed based on the pGreenII 62-SK vector. NtCYS promoter and the mutant promoter were cloned into the Sal I and Nco I site of the pGreenII 0800-LUC vector, respectively. The full length of NtCRF1 CDS was cloned into the Xba I and Kpn I site of the pGreenII 62-SK vector. The protoplasts were isolated from mesophyll cells of N. benthamiana . The plasmids were transfected into the protoplasts followed by 16 h incubation in the dark at 25 °C. The enzyme activity was measured using Dual-Luciferase® Reporter Assay System (E1910; Promega) in a microplate reader Biotek® Cytation3. Four independent measurements were carried out for the analysis. Quantification of endogenous GAs For determination of endogenous gibberellin in the seeds at stage −1, −3, and −5, we collected and grinded 500 mg seeds into powder as one sample after quick freezing with liquid nitrogen. Each sample was extracted with 5 ml of 90% aqueous methanol (MeOH) and 2 ng of each D-labeled GA compound as internal standards. The MAX cartridge (Waters) was activated and equilibrated with 10 ml MeOH, water, 5% NH 4 OH, and 90% MeOH in turn, while MCX (Waters) with 10 ml MeOH, water and 90% MeOH in order. Then the MAX cartridge was disconnected and washed with 5% NH 4 OH in 5% MeOH, MeOH successively. Finally, GAs were eluted with 2% formic acid in 90% MeOH. After dried with N 2 stream, the eluent was reconstructed with 200 μl 80% MeOH and subjected to UPLC-MS/MS analysis. GAs analysis was performed on a quadrupole linear ion trap hybrid mass spectrometer (QTRAP 5500, AB SCIEX) equipped with an electrospray ionization source coupled with a UPLC (Waters). Five microliter of each sample was injected into a BEH C18 column. GAs were detected in negative multiple reaction monitoring (MRM) mode. Each GA compound was quantified with a MRM transition and qualified with another one. 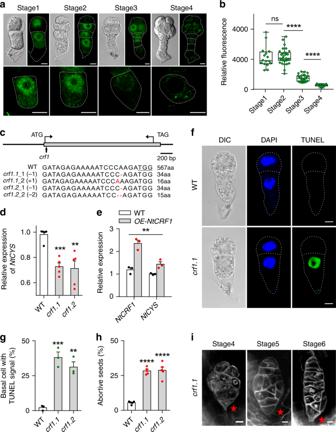Fig. 2 NtCRF1 promotesNtCYSexpression and suppresses PCD in basal cells.aLocalization of NtCRF1-GFP during early embryogenesis inpNtCRF1::NtCRF1-GFPplants. Magnified images of corresponding basal SCs are shown below.bRelative fluorescence intensity of NtCRF1-GFP in basal SCs (n= 16–31).cCRISPR/Cas9-mediated targeted mutagenesis ofNtCRF1. Top: Schematic ofNtCRF1showing the CRISPR/Cas9 target site (arrow). Bottom: Alignment of the sequences showing the insertion or deletion sites (red); numbers, translated amino acids (aa).dExpression ofNtCYSwas reduced in thecrf1mutants.eExpression ofNtCYSis increased in thepNtCRF1::NtCRF1-GFPline (OE-NtCRF1). (Two-way ANOVA, **P< 0.01).fNuclear DNA fragmentation in two-celled proembryos of WT andcrf1.1.gFrequency of two-celled proembryos with TUNEL-positive basal cells in WT andcrf1(n= 98–109).hFrequency of aborted seeds in WT andcrf1lines (n= 200–300 seeds per line).iAbnormal suspensors (stars indicated) incrf1lines by modified pseudo-Schiff-propidium iodide (PI) staining. Data are the means ± SE of 3 independent experiments ine,gand 5 independent experiments ind,h(Student’st-test, *P< 0.05, **P< 0.01, ***P< 0.001). Scale bars: 10 μm (a,f), 20 μm (i). The source data of the graphs are provided in the Source Data file Three independent samples were analyzed for each stage. Identification of NtGA3ox genes We firstly found GA3ox3 according the reference Ntab-TN90 Primary Assembly (BioProject: PRJNA319578) and its GO (Gene Ontology) annotation is ‘gibberellin 3-beta-dioxygenase 4-like’. Except two known GA3oxs , we found five annotated GA3ox -like genes in N. tabacum (Supplementary Fig. 11a ). 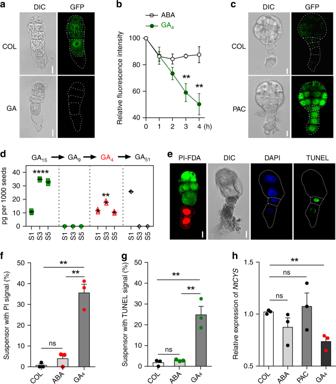Fig. 3 GA induces suspensor PCD via the NtCRF1-NtCYS pathway in vitro.aNtCRF1-GFP fluorescence in response to GA4in four-celled proembryos. 0.05% ethyl alcohol as control.bNtCRF1-GFP fluorescence in the basal cells of two-celled proembryos during treatment with GA4(or ABA) (n= 9).cNtCRF1-GFP in embryos derived from two-celled proembryo in cultured seeds after 72-h treatment with PAC.dQuantification of GA15, GA9, GA4, and GA51in WT seeds at stages 1, 3, and 5 (pg per 1000 seeds, ± SE).eCultured embryos stained with fluorescein diacetate (FDA), PI, and TUNEL.fFrequency of cultured embryos with PI-positive basal cells (n= 128–152).gFrequency of treated cultured embryos with TUNEL-positive basal cells (n= 106–126).hqRT-PCR analysis ofNtCYSexpression in 4-DAP seeds after treatment for 12-h with 100 μM ABA, PAC, or GA4. Data are the means ± SE of three independent experiments (Student’st-test; ns,P>0.05; **P<0.01; ****P< 0.0001). Scale bars: 10 μm. The source data of the graphs are provided in the Source Data file By sequence analysis, we chose the four of them for further analysis since the sequence of another one is distinctive compared to GA3oxs (Supplementary Fig. 11b ). We tested the six GA3oxs and found three of them ( NtGA3ox -1, -2, and -3) expressed in seeds before suspensor PCD. Thus, NtGA3ox -1, -2, and -3 were used for further analysis. Embryo isolation and seed clearing For embryo isolation, seeds were first treated in enzyme solution (1% cellulase R10, 0.5% macerozyme R10, 10.5% mannitol, and 3 mM MES, pH 5.5) for 30 min in the dark. Then droplets of the seed suspension were gently grinded by a flat-headed glass rod. After grinding several droplets of 10.5% mannitol were added for releasing and washing embryo sacs. Living embryos could be further isolated by a second enzymatic maceration procedure followed by a brief micromanipulation. For seed clearing, whole seeds were collected in a 2ml-centrifuge tube and were fixed by 50% methanol and 10% acetic acid at 4 °C for 12-h and then subjected to an overnight treatment of 1% SDS and 0.2 M NaOH at room temperature. Thereafter, the seeds were rinsed in water, followed by an incubation in 2.5% NaClO for 1-h, and then rinsed again. Next, the seeds were transferred into 1% periodic acid for 1-h at room temperature and in 80% ethanol for 10 min at 80 °C. Subsequently, the seeds were transferred back to the same fixative and incubated for 1-h before the seeds were rinsed again with water. After washing, the seeds were incubated in Schiff reagent with propidium iodide (PI) (P4170; Sigma) (100 mM sodium metabisulphite and 0.15 M HCl; PI to a final concentration of 0.1 mg/ml) for about 3-h. The samples were stored in a chloral hydrate solution (4 g chloral hydrate, 1 ml glycerol, and 2 ml water) and kept overnight at room temperature. Next, the chloral hydrate was replaced by Hoyer’s solution (30 g gum arabic, 200 g chloral hydrate, 20 g glycerol, and 50 ml water). The seeds were kept in the Hoyer’s solution for at least 10 days before observation under a confocal microscope. RNA-seq and data analysis mRNA of isolated two-celled proembryos (40–50 embryos per sample) was directly extracted using Dynabeads mRNA DIRECT TM Micro Kit (Life Technology). cDNA preparation was performed using the SMARTer Ultra Low Input RNA Kit for Sequencing v3 (Clontech). Libraries were constructed using TruePrep TM DNA Library Prep Kit V2 for Illumina (Vazyme) and then sequenced on Illumina HiSeq TM 4000. Adapters and low-quality reads were filtered using Cutadapt and an in-house script. Next, clean reads were mapped to the tobacco genome ( N. tabacum genome reference, Ntab-TN90) using Bowtie 2. Gene expression levels were quantified as FPKM (fragments per kilobase of transcript per million mapped reads) using RSEM. The raw data for each sample are available in the NCBI Gene Expression Omnibus under accession number GSE133373 . Cell viability and DNA fragmentation analyses To evaluate cell viability and plasma membrane integrity, we stained embryos with fluorescein diacetate (FDA) (F7378; Sigma) and PI. Isolated embryos were incubated in the solution containing 10.5% mannitol, 2 µg/ml FDA, and 1 µg/ml PI for 15 min at room temperature and washed twice with 10.5% mannitol before observation. To detect nuclear DNA fragmentation, the isolated embryos were tested by DeadEnd TM Fluorometric TUNEL System (G3250; Promega) or In Situ Cell Death Detection Kit, TMR red (12156792910; Roche) for pNtCRF1::NtCRF1-GFP line according to the manufacturer’s instructions, respectively. Two-celled proembryo culture in vitro The ovaries were rapidly surface-sterilized with 75% alcohol, followed by 5-min washes in sterile water for three times. Seeds were then isolated from the ovaries and collected in 2 ml 13% mannitol for co-culture. The isolated two-celled proembryos were transferred into a Millicell (PICM01250; Millipore) containing 100 μl of the medium [16] . The Millicell was put in a 3-cm Petri dish containing 1.5 ml of the medium [16] , and 100–150 seeds were co-cultured as feeder at 25 °C in the dark. 1 μM GA 4 or 1 μM ABA (A1049; Sigma) were added to the medium as appropriate. PAC, GA, ABA, and ethyl alcohol treatment assays Two-celled or four-celled proembryo isolated form pNtCRF1::NtCRF1-GFP line and treatment with 100 μM GA 4 for hours, 0.05% ethyl alcohol as control. Embryos derived from in cultured seeds form pNtCRF1::NtCRF1-GFP line after 72-h treatment with 100 μM PAC, 0.05% ethyl alcohol as control. 4-DAP WT seeds treated with 100 μM ABA, PAC (46046; Sigma), or GA 4 for 12-h, 0.05% ethyl alcohol as control, then collected for qRT-PCR. Quantitative real-time PCR Total RNA was extracted from leaves, roots, stems, anthers, sepals, and seeds using the MiniBEST Plant RNA Extraction Kit (9769; Takara). Total RNAs were treated with RNase-free DNase I (Promega), and cDNA was synthesized using Transcriptor Reverse Transcriptase (Invitrogen) according to the manufacturer’s instructions. 0.2 μl of resulting first-strand cDNA was used as a PCR template for qRT-PCR. 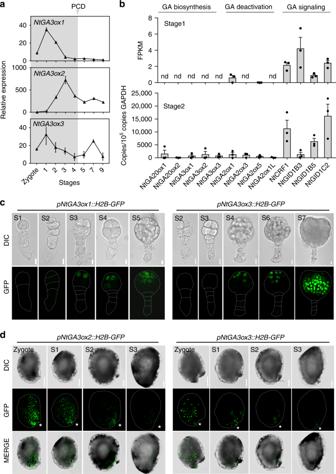Fig. 4 Bioactive GA biosynthesis during early embryogenesis.aqRT-PCR analysis ofNtGA3ox1,NtGA3ox2andNtGA3ox3expression;GAPDHwas used as the internal control.bExpression of genes related to GA biosynthesis [NtGA20ox1(Ntc12, AB012856.1) andNtGA20ox2(Ntc16, AB016084.1)], deactivation [NtGA2ox1(AB125232.1),NtGA2ox1-like(XM_016586923.1),NtGA2ox3(EF471117), andNtGA2ox5(EF471118)], and signaling in WT two-celled proembryos (stage 1) via transcriptome analysis, and via qRT-PCR analysis in WT four-celled proembryos (stage 2).GAPDHwas used as the internal control. Values are means ± SE of three biological replicates. nd, not detected.cExpression ofNtGA3ox1andNtGA3ox3during embryogenesis.dExpression ofNtGA3ox2andNtGA3ox3in the developing seed coat. Asterisks, micropylar ends; Scale bars: 10 μm (c), 100 μm (d). The source data of the graphs are provided in the Source Data file Quantitative PCR analysis were performed using FastStart Universal SYBR Green Master (4913850001; Roche) with a CFX Connect TM Real-Time System (Bio-Rad). Glyceraldehyde-3-phosphate dehydrogenase ( GAPDH ), or both GAPDH and Ubiquitin-conjugating enzyme2 ( UBI ) were used as the internal reference(s) to normalize the relative level of each transcript. Each experiment was repeated three or five times and each time the experiment included duplicate samples. The qPCR primer sequences are listed in Supplementary Data 1 . The raw data are shown in Source Data file. Transformation of BY-2 cells About 4 ml of 1-week-old tobacco BY-2 culture was first transferred into a 60-mm × 15-mm Petri dish, and then 20 μl prepared Agrobacterium tumefaciens line GV3101, containing p35S::NtCRF1-GFP or p35S::(crf1-Δ17)-GFP , was added into the culture dishes, respectively. Then each plate was sealed with Parafilm and incubated for 3-day at 28 °C in the dark on a shaker at 100 r.p.m. Subsequently, the cultured cells were washed four times and dipped in NT1 medium [34] containing 250 mg/L carbenicillin for 30 min to kill Agrobacterium, and then plated onto solid NT1 medium containing 250 mg/L carbenicillin and 50 mg/L kalamycin. After about 30-day, kalamycin-resistant calli appeared on the medium, and subsequently they were transferred onto new plates and suspended again in 50 ml liquid NT1 medium for observation. The cells were treated with 100 μM GA 3 for 4-h and 0.05% ethyl alcohol as control. The primers used are shown in Supplementary Data 1 . Confocal microscopy and image analysis Stained embryos were observed under a confocal microscope (Leica SP8). The nlsGPS1 emission ratio was determined as described [18] . Images were processed using ImageJ or Adobe Photoshop CC. Quantification and statistical analysis The fluorescence intensity was calculated as: integrated density—(area of selected cell nucleus × mean background fluorescence). 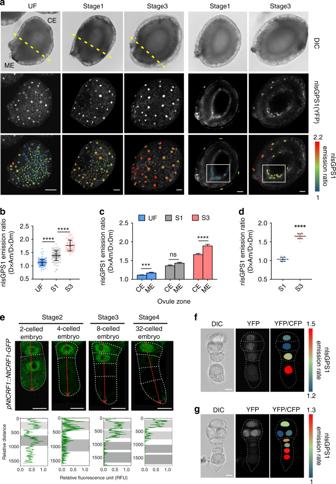Fig. 5 Transient increase in, and polar distribution of, bioactive GA in seeds.aLeft: Images of the nlsGPS1 emission ratios of unfertilized (UF), 4-DAP and 6-DAP seeds. Right: Images of the nlsGPS1 emission ratios of an optical section of a 4-DAP or 6-DAP seed. Boxes: micropylar endothecium.bBox plot of the nlsGPS1 emission ratios of the whole seed coat (n> 46 nuclei).cnlsGPS1 emission ratios of the micropylar and chalaza ends [dashed lines ina;n> 20 nuclei].dBox plot of the nlsGPS1 emission ratios of stage 1 or 3 seeds [boxed region ina;n> 10 nuclei].eNtCRF1-GFP was absent from the basal SC at stage 3. Fluorescence signal intensities along a line across all SCs (red arrows).X-axis, relative GFP signal intensity (green);y-axis, relative distances along the line. Gray shading, positions of nuclei.fandgImages of the nlsGPS1 emission ratios of 4-celled and 12-celled proembryos in WT background. Data are the means ± SD (standard deviations) (Student’st-test; ns,P> 0.05; ***P< 0.001; ****P< 0.0001). ME micropylar end, CE chalaza end. Scale bars: 100 μm (a), 10 μm (e–g). The source data of the graphs are provided in the Source Data file 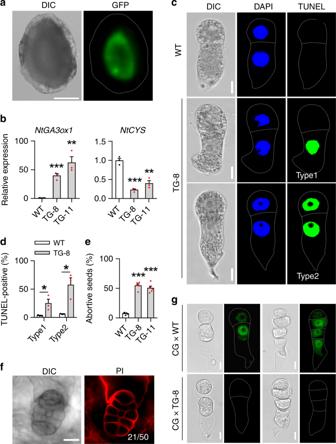Fig. 6 Ectopic expression ofNtGA3ox1-GFPin the endothelium triggers PCD.aLocalization of NtGA3ox1-GFP in the endothelium ofpNtTPE8::NtGA3ox1-GFPplant.bIncreased expression ofNtGA3ox1and decreased expression ofNtCYSin the TG-8 and TG-11 lines.cTUNEL test in two-celled proembryos from WT and TG-8.dFrequency of two-celled proembryos with TUNEL-positive apical and basal cells in WT and TG-8 (n= 105–112).eFrequency of aborted seeds in WT and TG-8. (n= 1000–1500).fPI-staining of abnormal embryos with no suspensor in the TG-8 line.gNtCRF1-GFP signal in early proembryos after crossing WT andpNtCRF1::NtCRF1-GFP(CG) lines. Data are the means ± SE of 3 independent experiments in (b,c) and 5 ine(Student’st-test, *P< 0.05, **P< 0.01, ***P< 0.001); Scale bars: 150 μm (a), 10 μm (c,g), 20 μm (f). The source data of the graphs are provided in the Source Data file qRT-PCR and fluorescence intensity data were assumed to follow normal distributions and were subjected to Student’s t -test or analysis of variance (ANOVA) using GraphPad Prism 7 software. The value of n , the definition of the center, dispersion, precision, and statistical significance are provided in the figure legends. * P < 0.05; ** P < 0.01; *** P < 0.001; **** P < 0.0001 compared to mock controls, unless otherwise specified by connecting lines. Reporting summary Further information on research design is available in the Nature Research Reporting Summary linked to this article.